Engineering the lymph node environment promotes antigen-specific efficacy in type 1 diabetes and islet transplantation Antigen-specific tolerance is a key goal of experimental immunotherapies for autoimmune disease and allograft rejection. This outcome could selectively inhibit detrimental inflammatory immune responses without compromising functional protective immunity. A major challenge facing antigen-specific immunotherapies is ineffective control over immune signal targeting and integration, limiting efficacy and causing systemic non-specific suppression. Here we use intra-lymph node injection of diffusion-limited degradable microparticles that encapsulate self-antigens with the immunomodulatory small molecule, rapamycin. We show this strategy potently inhibits disease during pre-clinical type 1 diabetes and allogenic islet transplantation. Antigen and rapamycin are required for maximal efficacy, and tolerance is accompanied by expansion of antigen-specific regulatory T cells in treated and untreated lymph nodes. The antigen-specific tolerance in type 1 diabetes is systemic but avoids non-specific immune suppression. Further, microparticle treatment results in the development of tolerogenic structural microdomains in lymph nodes. Finally, these local structural and functional changes in lymph nodes promote memory markers among antigen-specific regulatory T cells, and tolerance that is durable. This work supports intra-lymph node injection of tolerogenic microparticles as a powerful platform to promote antigen-dependent efficacy in type 1 diabetes and allogenic islet transplantation. The adaptive immune response provides antigen-specific protection against foreign pathogens while preserving tolerance against self-tissue. However, tolerance breaks down during autoimmune diseases such as type 1 diabetes (T1D), where pancreatic islets are targeted and destroyed. While T1D can be managed with frequent insulin administration, multiple comorbidities exist including cardiovascular [1] and gastrointestinal disease [2] . There are currently no approved therapies targeting the underlying immunopathology of T1D. Existing clinical therapies for autoimmune disease aim to restrain inflammation and self-reactivity using systemic administration of immunosuppressive drugs or modulatory therapies [3] . These treatments are not curative and require life-long compliance. Even the newest monoclonal antibodies do not distinguish between healthy and self-reactive cells, leading to serious side effects and non-specific immunosuppression [4] . For example, a monoclonal antibody targeting CD3—which suppresses and depletes effector T cells [5] —has delayed the loss of insulin production in patients previously diagnosed with T1D. This drug was recently demonstrated as the first immunotherapy in a clinical trial to significantly delay progression in at-risk T1D patients [6] , [7] . While more specific than classical immunosuppressants, this treatment is not curative and cannot distinguish healthy and autoreactive T cells. Another therapeutic approach for T1D is the transplantation of allogenic islets to restore control of insulin. However, these grafts are allogeneic, resulting in an attack by the recipient (i.e. host) T and B lymphocytes [8] , [9] . This requires nonspecific systemic immunosuppression to ameliorate graft rejection [10] . Novel treatments with molecular specificity are needed to address these persistent unmet clinical challenges. An experimental therapeutic concept in autoimmune disease is the induction of tolerance against specific self-antigens, without inhibiting normal adaptive immune responses needed to fight infection [11] , [12] . This strategy involves the administration of vaccine-like treatments that co-deliver relevant autoantigens with regulatory immune cues to redirect autoantigen-specific T cells toward populations with regulatory immune functions [13] , [14] , [15] , [16] , [17] , [18] , [19] , [20] . A number of these approaches focus on generation of regulatory T cells (T REG ), which exhibit potent tolerizing capabilities [21] . Because the fate of T cells during antigen encounter depends on signal integration in lymph nodes (LNs)—tissues that coordinate immunity [22] —a challenge of this approach is ensuring self and regulatory cues are presented in appropriate combinations and concentrations in LNs. Recently, intra-lymph node ( iLN) injection of soluble vaccines have shown promise in allergy [23] , [24] , cancer [25] , [26] , and T1D [27] , [28] . In these therapeutic contexts, i.LN injection has demonstrated striking potency and dramatic dose sparing in early trials [25] . While these trials utilized soluble signals which quickly drain from LNs, we’ve developed a system which employs i.LN injection of immune signals encapsulated in microparticle (MP) depots which are synthesized to be diffusion-limited and too large to drain out of LNs [29] . Instead, the MPs slowly degrade, locally concentrating immune cues that condition the local LN environment to direct immune cell fate. We have previously applied our modular i.LN platform to directly deposit antigens and modulatory immune cues, such as rapamycin (Rapa)—an inhibitor of the mammalian target of rapamycin (mTOR) pathway—in LNs to combat immune-mediated neurodegeneration during multiple sclerosis [30] . This work revealed i.LN treatment promoted tolerance in tandem with an increase in polyclonal T REG. However the effect of i.LN treatment on antigen-specific response has not been explored mechanistically. There are key questions that remain unknown with this platform, including the distinct roles of antigen and Rapa towards promoting a durable tolerogenic T cell response, how these immune signals affect structure of treated and untreated LNs is unknown, and lastly, whether this approach promotes tolerance or suppression in models of autoimmunity or alloimmune response driven by T cell responses against multiple antigens. To answer these questions, here we leverage our i.LN platform to directly study how immune cues impact the local LN microenvironment during antigen-specific autoimmunity in treated and untreated nodes in autoimmune and alloimmune disease models. We hypothesized application of this LN targeted approach to T1D and islet transplantation could obviate the need to administer high systemic doses of immunosuppressants through localizing tolerizing signals in LNs for tunable times and concentrations. Here we have applied this system to two distinct T1D contexts: pre-clinical models of CD4 and CD8-mediated T1D, and an allogenic islet transplant model in which full MHC mismatched donor islets are transferred to recipients after islet depletion. We synthesized MPs co-encapsulating Rapa and three distinct peptide antigens targeted in T1D or allograft rejection. In both models, MP formulations with appropriate antigens effectively prevented disease, and co-encapsulation of self-antigen with Rapa was critical for optimal protection in each case. MP treatment expanded antigen-specific T REG in treated and untreated LNs, and resulted in structural reorganization of LNs with microdomains associated with induction of tolerance. Finally, antigen-specific T REG displayed markers of enhanced persistence, and a single MP treatment stopped disease progression even when disease was induced at an extended timepoint following treatment. In contrast to all existing therapies which are administered systemically, local LN engineering could provide selective suppression or tolerance for autoimmune and alloimmune diseases without broad exposure to potent immunosuppressants (Fig. 1 ). Fig. 1: Overview schematic of iLN microparticle depot strategy to promote tolerance in T1D and allogenic islet transplantation. Intra-lymph node ( iLN ). This figure was created with Biorender.com. Full size image Tolerogenic MPs promote antigen-specific regulatory responses across multiple T1D-relevant self- and allo-antigens We hypothesized iLN depots could promote antigen-specific tolerance against pancreatic autoantigens and donor allo-antigens attacked on islets. Because in the NOD model of T1D tolerance can span multiple epitopes, we further hypothesized our platform would enable different antigens to be used interchangeably to drive tolerance across key epitopes underpinning T1D pathology. To test this, we selected NOD models of T1D where T1D can be induced by transfer of islet reactive T cells. Transgenic T cell receptor (TCR) mice with a NOD background have been engineered to express CD8 or CD4 T cells that are reactive to islet auto-antigens, and can be activated by mimotopes of islet peptide antigens. NOD8.3 TCR transgenic mice express CD8 TCRs which can be activated by the NRP-V7 [31] , [32] , [33] mimotope, and BDC2.5 transgenic mice express CD4 T cells that can be activated by the p31 [34] , [35] , [36] mimotope. For islet transplantation, we selected a full MHC mismatched islet transplant model using only one of the many I-E d class II MHC (EA) disparities to redirect the allogeneic response from immunity to suppression (Fig. 1 ). Poly(glycolide-co-lactide) (PLGA) MP depots were synthesized co-encapsulating Rapa with each self- (i.e., NRP-V7, p31) or allo-antigen (i.e., Ea) (Fig. 1 ). 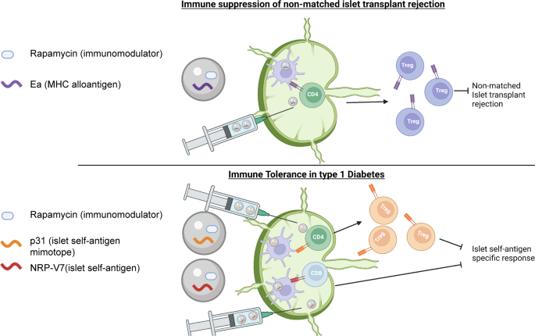Fig. 1: Overview schematic ofiLNmicroparticle depot strategy to promote tolerance in T1D and allogenic islet transplantation. Intra-lymph node (iLN). This figure was created with Biorender.com. MP properties for each formulation are listed in Supplementary Table 1 . In co-cultures consisting of DCs from NOD mice and T cell receptor transgenic CD4 T cells from BDC2.5 transgenic mice that recognize p31 antigen presented by DCs, p31/Rapa MP partially inhibited T cell proliferation compared to p31 (Fig. 2a, b ). However, phenotypic analysis of the expanding BDC2.5 T cells revealed p31/Rapa MP significantly increased T REG frequency (Fig. 2c, d , Supplementary Fig. 1a ). This polarization was also associated with decreased production of T H 1- and T H 17-associated inflammatory-cytokines IFNγ (Fig. 2e, f ) and IL-17 (Fig. 2g, h ), respectively. Analogous shifts from inflammation to tolerance (i.e., T REG ) were observed during co-culture of DCs with TEa transgenic CD4 T cells treated with Ea/Rapa MPs, but not Ea MPs (Fig. 2i–k ). Since almost no endogenous T REG are present in TEa mice, Ea/Rapa MPs promote a TEa T REG response through conversion of non-T REG (Supplemental Fig. 2a, b ). Lastly, during co-culture of DCs and NOD8.3 CD8 T cells, NRP-V7/Rapa MP significantly restrained proliferation (Fig. 2l ) and IFNγ production (Fig. 2m, n , Supplementary Fig. 1b ). Together these data demonstrate antigen-specific tolerization and control of inflammation in three distinct T1D contexts that span self- and alloantigen, as well as CD4- (i.e., BDC2.5, TEa) and CD8-driven (i.e., NOD8.3) inflammatory T cells. Fig. 2: MPs encapsulating relevant antigens and Rapa promote suppressive T cell responses in vitro. BDC2.5 T cell co-cultures were treated with p31 MP or p31/Rapa MPs. a Quantification of BDC2.5 T cell proliferation and b representative flow cytometry plots of CSFE dilution are shown. c Quantification of Foxp3 expression and d representative flow cytometry plots are shown. e Quantification of IFNγ expression and f representative flow cytometry plots are shown. g Quantification of IL-17 expression and h representative flow cytometry plots are shown. TEa T cell co-cultures were treated with Ea MP or Ea/Rapa MPs. Quantification of i proliferation, j Foxp3 expression and k IFNγ expression are shown. NOD8.3 T cell co-cultures were treated with NRP-V7 MP or NRP-V7/Rapa MPs. l Representative flow cytometry plots showing proliferation and quantification of m proliferation and n IFNγ production are shown. N = 3 individual culture wells for all experiments. Plots represent mean ± s.d. One-way ANOVA with Tukey’s post test used to compare treatment groups and comparisons between matched doses of p31 and p31/Rapa MPs are shown. * p < 0.05, ** p < 0.01, *** p < 0.001, **** p < 0.0001. Source data are provided as a Source Data file. Full size image Direct LN injection of tolerogenic MPs promotes tolerance in pre-clinical models of T1D and islet transplantation As an initial setting to test the tolerizing ability of MPs in T1D, we used an accelerated model of T1D where ex vivo activated NOD8.3 T cells are adoptively transferred into NOD mice (Fig. 3a ). Mice were treated iLN (Supplemental Fig. 3 ) 3 days prior to T cell transfer to test if NPR-V7/Rapa MPs could inhibit T1D, and importantly, if MPs loaded with a different disease-relevant peptide (i.e., p31/Rapa MPs) could also prevent disease. Excitingly, a single treatment of either NRP-V7/Rapa MP or p31/Rapa MPs prevented disease in all animals, whereas p31-only MPs provided no benefit relative to the vehicle (Fig. 3b, c ). These data indicate the inclusion of either a CD4-dominant (p31) or CD8-dominant (NRP-V7) epitope provided efficacy, even when the disease was mediated by CD8 reactivity (i.e., NOD8.3 TCR transgenic T cells). We also note Rapa MPs partially inhibited disease, which may have resulted from nonspecific transient suppression. To benchmark iLN MPs against a conventional treatment formulation and route, mice were treated iLN with p31/Rapa MPs or i.p . with free p31 and Rapa 3 days before adoptive transfer of NOD8.3 T cells (Supplemental Fig. 4a ). iLN provided significant efficacy compared to i.p treatment of free p31 and Rapa (Supplemental Fig. 4b, c ). In studies discussed later, we employed additional regimens to further investigate the role of each component and the durability of induced tolerance. Future studies will focus on testing the ability of iLN p31/Rapa MPs to inhibit disease in the spontaneous NOD model of T1D. Fig. 3: iLN injection of tolerogenic MPs promotes tolerance in T1D and suppression of graft rejection in allogenic islet transplantation. a Schematic representation of prophylactic iLN treatment in the NOD8.3 model of T1D. b Survival curve with number of mice which developed disease out of the total mice per group indicated in the parenthesis in the legend. c Individual blood glucose traces for mice in each group from b . d Schematic representation of iLN treatment in the non-matched islet transplant model. e Survival curve for experiment detailed in d . f Individual blood glucose traces for mice in each group ( d ). N = 5 mice for all groups except N = 4 mice for Rapa MP treatment group. Two-tailed log-rank (Mantel-Cox) was used for all pairwise comparisons between each treatment for survival curves in b . * p < 0.05, ** p < 0.01, *** p < 0.001, **** p < 0.0001. Source data are provided as a Source Data file. Intra-lymph node ( iLN ), streptozotocin (STZ). Full size image We next tested the ability of iLN MPs to inhibit islet allograft rejection in a full MHC mismatched transplantation model. Islets were chemically depleted in C57BL/6 mice using streptazotocin (STZ), followed by transplantation of allogeneic islets from BALB/c mice underneath the kidney capsule (Fig. 3d ). In this model, alloantigen of donor islets is targeted by the host adaptive immune response. iLN treatment was administered once on the first day of the disease, determined by hyperglycemia. For peptide antigen to induce suppression, we chose only a single I-E d α-chain disparity between donor and recipients, leaving untargeted a multitude of other MHC class I and minor antigen differences between the two mouse strains. Vehicle, Empty MP, and Ea MP treated cohorts all rapidly rejected transplanted islets (Fig. 3e, f ), with median survivals of 9, 12 and 11 days, respectively. Similar to the NOD8.3 model, Rapa MP alone modestly prolonged survival compared to Vehicle or MPs encapsulating Ea antigen alone. Intriguingly, Ea/Rapa MPs provided significant therapeutic benefit with a median survival of 56 days vs 21 days and 9 days for Rapa MPs and vehicle, respectively (Fig. 3e, f ). While Ea/Rapa MPs dramatically prolonged survival in the islet transplantation model, they were unable to fully restore tolerance unlike p31/Rapa MPs or NRP-V7/Rapa MPs in the T1D model. This difference in efficacy may be due to the much stronger immune response induced against the multitude of alloantigens targeted in the full MHC mismatched transplantation model. Future experiments will investigate if co-delivering multiple alloantigens with Rapa can more effectively suppress this broad alloimmune response. This approach could offer broader, personalized-like tolerance, or dose sparing. Together, efficacy in these pre-clinical models reveals depots potently combat T1D and islet rejection with one treatment, and co-encapsulation of Rapa and disease-relevant—but not necessarily disease-induction—epitope maximize efficacy. p31/Rapa MPs prime antigen-specific T cells in treated and untreated LNs while suppressing mTOR activity Since MP treatment promotes tolerance with respect to disease pathology, we next investigated the mechanism and localization of T cell polarization by testing if MPs prime antigen-specific T cells and inhibit mTOR in treated and untreated LNs. NOD mice were injected with p31/Rapa MPs in the inguinal LNs, then BDC2.5 T cells were adoptively transferred to ensure a large population of antigen-specific T cells for analysis (Fig. 4a ). BDC2.5 T cells were labeled with CSFE prior to cell transfer to allow tracking at early timepoints. One day after transfer we isolated the transferred cells from LNs (Fig. 4b ) and analyzed them for CD69 and phosphorylated ribosomal s6 protein (ps6) expression. CD69 is an early activation marker upregulated within hours of antigen-specific stimulation, while ps6 correlates with increased mTOR signaling. BDC2.5 T cells in treated LNs of mice receiving MP formulations containing p31 antigen (i.e., p31 with or without Rapa) displayed similar levels of CD69 expression, which were elevated compared to cells in treated LNs of mice receiving MP formulations without antigen (Fig. 4c, d , Supplementary Fig. 5a ). Interestingly, this trend was also observed in the untreated axillary LNs, which drain the treated inguinal LNs at early timepoints, and to a lesser extent in the pancreas-draining LNs and the distant later-draining popliteal LNs (Fig. 4c, d ). These data suggest the systemic presentation of either the p31 peptide or endogenous autoantigen. Concurrently with the upregulation of early activation markers, we discovered inclusion of Rapa in MPs dramatically suppressed phosphorylation of s6 through the mTOR pathway within these cells (Fig. 4e, f , Supplementary Fig. 5b ). Once again, this trend was present in treated and untreated LNs. Together these data demonstrate p31/Rapa MPs prime antigen-specific T cells and modulate mTOR activity, a combination of features that we hypothesized could provide sufficient stimulus for T cell expansion, while polarizing these self-specific cells toward T REG . Fig. 4: p31/Rapa MPs promote antigen-specific T cell priming while inhibiting mTOR in vivo. a Schematic representation of MP treatment and experimental readout for BDC2.5 T cell adoptive transfer experiment. b Illustration of lymph nodes collected and their anatomical relevance to treatment. c Representative flow cytometry traces and d quantification of CD69 expression among p31 specific T cells. e Representative flow cytometry traces of phosphorylated s6 among CD69 + p31 specific T cells in treated LNs and f quantification in all LNs. N = 4 mice for all experiments, and paired LNs (i.e. inguinals, axillary, popliteal) were pooled for each mouse. The mean ±; s.d. is shown. One way ANOVA with Tukey’s post hoc test was used to compare each treatment within individual lymph nodes. * p < 0.05, ** p < 0.01, *** p < 0.001, **** p < 0.0001. Source data are provided as a Source Data file. Intra-lymph node ( iLN ), phosphorylated ribosomal s6 protein (ps6). Full size image MPs expand antigen-specific T REG in treated and untreated LNs To investigate further the above-mentioned hypothesis, we tested if MP treatment expands antigen-specific T REG by again treating NOD mice iLN with MPs and transferring CSFE labeled BDC2.5 T cells (Fig. 5a ). Two and seven days after T cell transfer, treated and non-treated LNs were isolated (Fig. 5b ). In this experiment T cells were from BDC2.5 mice with a Thy1.1 syngeneic marker. This was used to enable tracking at later timepoints when CSFE dilution due to proliferation makes it overwise impossible to distinguish transferred and host cells. At 2 days post transfer—while both p31 MPs and p31/Rapa MPs induced BDC2.5 T cell proliferation (Fig. 5c, d , Supplementary Fig. 6 ), the frequency of proliferated cells was significantly higher in the treated, early-draining, and pancreatic LNs (untreated) of mice treated with p31 MP relative to p31/Rapa MP treatment (Fig. 5d ). Seven days post transfer, nearly all BDC2.5 T cells in mice treated with p31 or p31/Rapa MPs had proliferated in each LN examined, including distant, later-draining LNs (Fig. 5c, e ). The total degree of proliferation was higher among T cells in mice treated with p31 MPs compared to p31/Rapa MPs in treated LN (Supplementary Fig. 7a–c ). However, in each case the frequency of proliferated T cells was significantly higher in p31 MP or p31/Rapa MP-treated mice compared to vehicle or Rapa MP-treated mice in each LN. At day 2, the total frequency of BDC2.5 T cells in LNs among all CD4 T cells was low (<0.5% for each group in each LN) (Fig. 5f ). By day 7, the frequency of BDC2.5 T cells increased in both treated and draining LNs of mice receiving p31/Rapa MPs and p31 MPs, but intriguingly, p31/Rapa MPs caused significantly greater increases than p31 MPs, representing a threefold expansion in treated LNs. (Fig. 5g ). Finally, while analysis of Foxp3 expression showed no differences among BDC2.5 T cells at day 2 in any LN (Fig. 5h, j ), by day 7, p31/Rapa MP treatment dramatically expanded T REG frequencies and numbers (Supplementary Fig. 7f ) among antigen-specific T cells in treated and the early-draining LNs compared to all treatment groups (Fig. 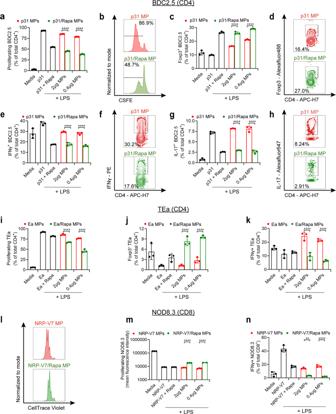Fig. 2: MPs encapsulating relevant antigens and Rapa promote suppressive T cell responses in vitro. BDC2.5 T cell co-cultures were treated with p31 MP or p31/Rapa MPs.aQuantification of BDC2.5 T cell proliferation andbrepresentative flow cytometry plots of CSFE dilution are shown.cQuantification of Foxp3 expression anddrepresentative flow cytometry plots are shown.eQuantification of IFNγ expression andfrepresentative flow cytometry plots are shown.gQuantification of IL-17 expression andhrepresentative flow cytometry plots are shown. TEa T cell co-cultures were treated with Ea MP or Ea/Rapa MPs. Quantification ofiproliferation,jFoxp3 expression andkIFNγ expression are shown. NOD8.3 T cell co-cultures were treated with NRP-V7 MP or NRP-V7/Rapa MPs.lRepresentative flow cytometry plots showing proliferation and quantification ofmproliferation andnIFNγ production are shown.N= 3 individual culture wells for all experiments. Plots represent mean ± s.d. One-way ANOVA with Tukey’s post test used to compare treatment groups and comparisons between matched doses of p31 and p31/Rapa MPs are shown. *p< 0.05, **p< 0.01, ***p< 0.001, ****p< 0.0001. Source data are provided as a Source Data file. 5i, k , Supplementary Table 2 ). In addition to T REG , p31-specific Foxp3 - T cells (non-T REG ) also proliferated in mice treated with p31/Rapa MPs (Supplementary Fig. 7a–d ). p31/Rapa MP treatment also increased T REG frequency among the total CD4 population compared to p31 MPs (Supplementary Fig. 7e ). Since BDC2.5 mice develop endogenous T REG [37] , the increased T REG frequency among transferred cells may be driven by p31/Rapa MP-induced maintenance or expansion of pre-existing natural or peripheral T REG , de novo generation of T REG , or conversation of conventional T cells. Future studies will explore these possibilities. Together these data demonstrate the presence of cognate antigen is required to expand antigen-specific T cells in treated and untreated LNs, and inclusion of Rapa is necessary to polarize antigen-specific T cells to T REG . Fig. 5: p31/Rapa MPs expand antigen-specific T REG in treated and untreated LNs. a Schematic representation of MP treatment and experimental readout for BDC2.5 T cell adoptive transfer experiment. b Illustration of LNs collected and analyzed. c Representative flow cytometry traces and quantification of p31 specific T cell proliferation at d day 2 and e day 7. Quantification of p31 specific T cell frequency at f day 2 and g day 7. Representative flow cytometry traces showing Foxp3 expression among p31 specific T cells in treated LNs at h day 2 and i day 7. Quantification of Foxp3 expression among p31 specific T cells at j day 2 and k day 7 in each LN analyzed. N = 5 mice for all groups in all experiments, and paired LNs were pooled for each mouse. The mean ±  s.d. is shown. For all comparisons in this figure between mice treated with different treatments, One-way ANOVA with Tukey’s post hoc test was done between all treatment groups within each individual LN. All comparisons between the Rapa MP and p31/Rapa MP treatment groups among different tissues were also done using One way ANOVA with Tukey’s post hoc test, and the p values from this analysis are listed in Supplemental Table 2 . * p < 0.05, ** p < 0.01, *** p < 0.001, **** p < 0.0001. Source data are provided as a Source Data file. Intra-lymph node ( iLN ). Full size image The release rate of antigen and Rapa may influence tolerance induction through modulating the dose and persistence of antigen and Rapa in LNs during T cell priming, thus impacting the magnitude and phenotype of the T cell response [38] . In vitro release studies demonstrated rapamycin and p31 were released over time from MPs, with p31 displaying more rapid release. 88 ± 5.1% of total encapsulated p31 was released and 18.4 ± 8% of total Rapa were released after 48 h (Supplementary Fig. 8 ). While MP formulations may be tuned in future studies to determine an optimum for promoting tolerance, in this study we utilized MPs formulated similarly to MPs employed in our previous studies where tolerance was achieved in mouse models of multiple sclerosis [30] . We found p31-specific T cells proliferated in injected LNs of mice treated with p31/Rapa MPs 3 weeks after MP injection, demonstrating prolonged antigen release and presentation following MP injection in vivo (Supplementary Fig. 9a , b ). Previous work in multiple models of autoimmune disease has demonstrated systemic delivery of antigen in particulate form in the absence of a regulatory cue can promote antigen-specific tolerance [12] , [18] , [39] , [40] , [41] , [42] , [43] . The mechanisms involved in these studies generally leverage antigen processing through non-inflammatory pathways by antigen-presenting cells (APCs) in LNs, spleens, and liver to restrain antigen-specific immune response. Presentation of antigen in these contexts results in functional deletion or exhaustion of auto-antigen-specific effector T cells and promotion of active tolerance through the generation of T REG . In contrast, iLN injection of MPs delivering antigen alone expands antigen-specific T cells, does not increase antigen-specific T REG (Fig. 5k ) and does not inhibit disease in T1D (Fig. 3b ) or islet transplantation (Fig. 3e ). These data suggest mechanistically self-antigen is not processed in a tolerogenic manner when delivered iLN alone, and instead provides necessary activation and expansion of antigen-specific T cells which are then polarized by Rapa to drive regulatory phenotype. Interestingly, iLN treatment with p31/Rapa MPs does not exhaust antigen-specific T cells but promotes active tolerance which may provide durable control of autoimmune reactions. Further study is needed to elucidate the exact role antigen-specific T REG play in promoting tolerance. Future studies will also investigate the interplay of expanded T REG and inflammatory T cell phenotypes such as T H 1 or T H 17. While the expanded non-T REG cells may have the potential for pro-inflammatory response, it is clear they are controlled in vivo, and the overall antigen-specific response is tolerogenic (Fig. 3b, e ). Antigen delivered in MPs is presented in treated and untreated LNs, with presentation in untreated LNs independent of APC migration The finding that after LN injection of MPs containing antigen, CD69—which is transiently upregulated upon stimulation and facilitates temporary retention in LNs [44] —is upregulated in both treated and non-treated LNs (including non-pancreas draining LNs) suggests antigen delivered in MPs is presented in these sites. Since these MPs are size restricted and do not drain through efferent lymphatics, there are two likely mechanisms for delivery to LNs: drainage through lymphatics after release from MPs or trafficking by APCs after internalization of MPs. To confirm MPs are retained in treated LNs, mice were injected iLN with unlabeled MPs, or MPs encapsulating a fluorescent dye, DiR (DiR MPs) (Fig. 6a ). 2 and 4 days after MP treatment, treated, early-draining and pancreatic-draining LNs were isolated and imaged by IVIS for DiR signal. No DiR signal was detected in any LNs receiving unlabeled MP formulations. However, there was significantly increased DiR signal in LNs treated with DiR MPs 2 days after treatment. In these groups DiR signal was only detectable in treated LNs, supporting local MP retention in treated LNs (Fig. 6b, c ). These data demonstrate the restriction of large cargo reservoirs to the treated LNs using intra-LN depots. Fig. 6: Ea is presented in treated and untreated LNs after Ea/Rapa MP treatment. a Schematic representation of experiment in panels b – d . b IVIS images of excised treated LNs. c Quantitation of DiR MP signal in excised LNs. Two-tailed Welch’s t test was used to compare both treatment groups within individual lymph nodes at each time point. Individual LNs were used as single data points. Mean ± s.d. is shown. N = 3 mice for DiR MP treatment groups and N = 1 mouse for empty MP treatment group at each timepoint. Each LN is represented as an individual data point. d Schematic representation of experiment in panels f – i . e Representative immunofluorescent images of LNs stained with ER-TR7, CD11c, YAe; Scale bar = 50 μm. Quantification of Ea presentation in MHC-II (YAe) in f treated, g early-draining and h late-draining LNs. N = 2 mice for each timepoint, with 2 or 3 sections per LN. One way ANOVA with Dunnett’s post hoc test was used to compare percent YAe area to the naive control at each timepoint. i Schematic representation of experiment in panels k – m . Quantification of Ea presentation in MHC-II in j treated, k early-draining and l late-draining LNs after FTY720 treatment. One-way ANOVA with Tukey’s post hoc test was used to compare each group. N = 2 mice for each timepoint, with 2 or 3 sections per LN. Mean ± s.d. is shown for each sample in each experiment. * p < 0.05, ** p < 0.01, *** p < 0.001, **** p < 0.0001. Source data are provided as a Source Data file. Intra-lymph node ( iLN ). Full size image To confirm antigen presentation in untreated LNs, we directly investigated the trafficking and presentation of antigen from MPs in untreated LNs using the Y-Ae mAb which directly recognizes the EA peptide when presented in by MHC class II of the recipients [45] . To study Ea presentation, mice were immunized iLN with Ea/Rapa MPs on day −1, then the treated and untreated LNs were stained for Ea presentation in areas of LNs surrounding high endothelial venules (HEVs) on days 0, 2, and 6 (Fig. 6d ) in the cortical ridge (CR) [46] . 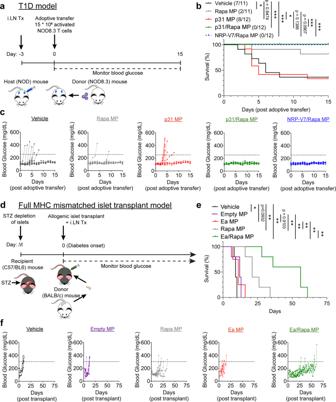Fig. 3:iLNinjection of tolerogenic MPs promotes tolerance in T1D and suppression of graft rejection in allogenic islet transplantation. aSchematic representation of prophylacticiLNtreatment in the NOD8.3 model of T1D.bSurvival curve with number of mice which developed disease out of the total mice per group indicated in the parenthesis in the legend.cIndividual blood glucose traces for mice in each group fromb.dSchematic representation ofiLNtreatment in the non-matched islet transplant model.eSurvival curve for experiment detailed ind.fIndividual blood glucose traces for mice in each group (d).N= 5 mice for all groups exceptN= 4 mice for Rapa MP treatment group. Two-tailed log-rank (Mantel-Cox) was used for all pairwise comparisons between each treatment for survival curves inb. *p< 0.05, **p< 0.01, ***p< 0.001, ****p< 0.0001. Source data are provided as a Source Data file. Intra-lymph node (iLN), streptozotocin (STZ). These regions create critical networks where antigens, APCs/DCs, and T cells interface to initiate and direct antigen-specific immune processes, including suppression and tolerance [47] , [48] . At 2 days, Ea presentation localized with HEVs was detected in treated LNs (Fig. 6e ), and increased by day 6 (Fig. 6f ). Likewise, at day 2, Ea presentation localized with HEV was also detected in the early-draining (Fig. 6g ) and late-draining (Fig. 6h ) LNs; by 6 days the signal in the late-draining LNs remained elevated (Fig. 6h ). Since antigen presentation was confirmed in untreated LNs after iLN injection, and MPs were restricted to treated LNs, we next tested if antigen trafficking may be through lymphatic drainage following release from MPs, or through migration of APCs that internalize MPs. Mice were immunized with Ea MPs or Ea/Rapa MPs, and then APC egress from LNs was inhibited by administration of FTY720 [49] —an antagonist of the S1P receptor—using three daily i.p . injections starting on the day of MP treatment (Fig. 6i ). 1 day after the final FTY720 injection, treated and draining LNs were analyzed for Ea presentation in HEVs. In every LN analyzed, Ea and Ea/Rapa MP treatment significantly increased Ea presentation in treated (Fig. 6j ), early-draining (Fig. 6k ) and late-draining LNs (Fig. 6l ) compared to the non-injected control. FTY720 treatment did not significantly affect Ea presentation (Fig. 6j–l ) by either MP treatment. This discovery suggests trafficking of antigen from MP-treated LNs to distant LNs is not reliant on migration of APCs from the treated LNs, and instead results from lymphatic drainage. Here we’ve demonstrated a single iLN injection promotes potent tolerance through concentrating delivered cargo in LNs. Such capabilities could provide significant potential for dose sparing compared to current systemic clinical regimens [50] , [51] . While the presentation of antigen without the presence of Rapa in untreated LNs has the potential to prime antigen-specific T cells with inflammatory function, the fact that iLN treatment with MPs encapsulating antigen alone does not significantly alter disease in T1D (Fig. 3b ), or allogenic islet transplantation compared to vehicle controls (Fig. 3e ) indicates activation of antigen-specific T cells with pro-inflammatory potential is not of significant concern. While biodistribution of Rapa after MP treatment requires further study, inhibition of mTOR signaling in untreated tissues of p31/Rapa MP treated mice (Fig. 5c, d ) likely indicates dissemination of Rapa to these LNs, similar to antigen. The concentrations of antigen and Rapa accumulating in untreated LNs, and their impact on the tolerogenic immune response is unclear. However, we have previously demonstrated the co-delivery of immunostimulatory adjuvants and antigen using the iLN platform with MPs promoted superior antigen-specific T cell response compared to treatment with LN nanoparticles (NPs) sufficiently small to drain through efferent lymphatics [29] . Therefore, we hypothesize prolonged retention of delivered cargo in treated LNs after MP treatment is the main driver for induction of tolerance. An additional key advantage of the iLN platform is the ability to deliver the entire dosage of immune signals to the lymphatic system in order to promote antigen-specific T REG in LNs without exposing peripheral tissue to high-dose immunosuppressants. While particulate delivery of antigen can enter the lymphatics and reach multiple LNs after peripheral administration, a large fraction of payload is retained at the injection site or can reach the non-lymphoid tissues depending on particle size and properties [38] , [52] . iLN microparticle delivery can improve these shortcomings. In these studies we have used a non-surgical technique to inject peripheral LNs which do not drain the pancreatic islets. It has been demonstrated that LNs differ in their propensity to promote tolerogenic or inflammatory T cell responses and to imprint T cell migratory potential based on their location and drainage patterns. Priming in skin draining LNs drives T cell migration to the skin via CCL10 expression [53] , while T cell priming in gut draining LNs drives T cell migration to the gut in a retinoic acid dependent manner [54] . A previous report has shown proximal gut draining LNs preferentially promote tolerogenic responses, where distal gut draining lymph nodes promote inflammatory responses toward the same antigen [55] . Therefore, future work should investigate whether selection of LN to inject will impact efficacy in promoting tolerance. In addition, future studies should investigate the ability of MP-induced antigen-specific T REG to migrate to the pancreatic islets following peripheral LN injection. In clinical settings it may be advantageous to inject islet-draining LNs when accessible during surgical islet transplantation. However, since antigen (Fig. 6e–h ) and most likely Rapa, as discussed above, disseminate to other LNs along with antigen-specific T REG (Fig. 5k ) after iLN MP treatment, non-surgical injection of peripheral LNs may provide similar efficacy while obviating the need for surgery and will allow for future boosts if needed. In fact, clinical trials utilizing iLN injections of free islet autoantigens have injected inguinal LNs non-surgically with ultrasound guidance [27] . LN delivery of MPs promote a tolerogenic LN microenvironment Using genetic knock out models, we have shown during tolerance, structural changes develop in LN stroma. These are characterized by increases in the ratio of laminin α4 (lama4) to laminin α5 (lama5) locally in the HEVs and CRs of LNs [45] , [56] , [57] . In these regions, higher lama4:lama5 ratio promotes T REG induction and accumulation, while lower ratios favor differentiation of T H 1 and T H 17 phenotypes [56] . Thus, we tested if local delivery of MPs containing self-antigen and Rapa promote tolerogenic microdomains and local T REG polarization in treated LNs. Mice were immunized with Ea/Rapa MPs followed by adoptive transfer of TEa T cells. One day after T cell transfer, treated LNs were analyzed for lama4 and lama5 expression in HEVs and CR (Fig. 7a , Supplementary Fig. 10a ). HEVs and CRs were identified based on morphology of the stromal fibers, ER-TR7, which are produced by fibroblastic reticular cells in CRs and encase HEVs [45] . In both HEVs (Fig. 7b, c , Supplementary Fig. 11a–c ) and CR (Fig. 7b, d , Supplementary Fig. 11d , e ), Ea/Rapa MPs promoted the highest lama4:lama5 ratio. In CRs Rapa MPs but not Ea MPs also significantly increased lama4:lama5 ratio, highlighting the modulatory cue as the key driver of structural rearrangement. Similar results were observed in NOD mice treated with p31/Rapa MPs and infused with BDC2.5 T cells (Fig. 7e ); lama4:lama5 ratios were significantly increased in HEVs when comparing p31/Rapa with p31 treatment (Fig. 7f ). These data demonstrate co-treatment with Rapa and antigen—either p31 or Ea, promotes local stromal changes in LNs associated with induction of T REG response. Fig. 7: MP treatment promotes development of tolerogenic microdomains in LNs. a Schematic representation of experiment in panels b – d . b Representative immunofluorescence images of treated LNs stained for laminin α4, laminin α5, ER-TR7, and DAPI are shown; Scale bar = 50 μm. Quantification of ratio of laminin α4 to laminin α5 in c high endothelial venules and d cortical ridges in treated LNs. N = 4 mice for each treatment group with 2 or 3 sections per LN. One-way ANOVA with Tukey’s post hoc test was used to compare treatment groups. e Schematic representation of experiment in panel f . f Ratio of laminin α4 to laminin α5 in high endothelial venules of LNs. N = 4 mice for each treatment group with 2 or 3 sections per LN. Two-tailed Welch’s t test was used to compare groups, and inguinal, axillary and pancreatic LNs were pooled for each treatment group. g Schematic representation of experiments in panels i – l . h Representative immunofluorescence images showing Foxp3 expression among antigen-specific T cells in treated LNs. The naïve group did not receive adoptive transfer of Ea T cells. DAPI (Blue) and ER-TR7 (Cyan) are included in the merge: Scale bar = 50 μm. LNs were stained for Foxp3, Vα4 T cell receptor clonotype, ER-TR7, and DAPI. Representative merged images are show in Supplementary Fig. 10 . Quantification of Foxp3 expression among antigen-specific T cells in i high endothelial venules (HEV) and j cortical ridges (CR). Quantification of ratio of laminin α4 to laminin α5 in k high endothelial venules and l cortical ridges in treated and untreated LNs. N = 4 mice for each treatment group with 2 or 3 sections per LN. Iliac LNs were used as untreated LNs. One-way ANOVA with Tukey’s post hoc test were used to compare each treatment group within individual lymph nodes in each region of the LN analyzed. For all experiments mean ± s.d. is shown. * p < 0.05, ** p < 0.01, *** p < 0.001, **** p < 0.0001. Source data are provided as a Source Data file. Intra-lymph node ( iLN ). Full size image To determine if iLN MP-induced stromal rearrangement promotes local accumulation of antigen-specific T REG in HEVs and CRs, C57BL/6 mice were immunized with Ea/Rapa MPs, followed by adoptive transfer of Ea TCR transgenic T cells. 3 days after T cell transfer, non-matched BALB/c donor-specific splenocytes (DST) exhibiting Ea were adoptively transferred i.v . to generate a systemic alloimmune response [45] . Two days following DST infusion, LNs were analyzed for T REG accumulation in HEVs and CRs (Fig. 7g ). To identify antigen-specific T REG , LNs were co-stained for Foxp3 and the Vα4 T cell receptor chain, which is expressed by the Ea T cells [45] . Ea/Rapa MPs promoted the greatest increase of antigen-specific T REG in HEVs and CRs (Fig. 7h–j , Supplementary Fig. 10b ). Interestingly, Rapa MP treatment did not promote TEa T REG despite increasing lama4:lama5 ratio in HEVs of treated and untreated LNs and CRs of treated LNs (Fig. 7k, l ). This is surprising since DST infusion provides a source of Ea antigen for TEa T cell priming in LNs. The necessity of delivering Ea in MPs to promote T REG accumulation may be explained by prolonged retention of Ea in LNs after MP delivery compared to DST. Together these data indicate cognate-antigen/Rapa MPs promote tolerogenic microdomains in LNs in both homeostatic and inflammatory conditions. Rapa MPs and antigen/Rapa MPs inhibit disease transfer in therapeutic treatment regimens, while co-delivery of antigen with Rapa is required to provide durable immunosuppression in the NOD8.3 model of T1D Since antigen/Rapa MPs completely inhibited disease in the NOD8.3 model when given 3 days before disease induction (Fig. 3 b), we next tested if iLN MP treatment could promote tolerance in a more challenging therapeutic regimen. In this regimen, mice were treated i.LN with MPs 1 day after T cell transfer (Fig. 8a ). Similar to the prophylactic treatment regimen (Fig. 3a–c ), p31/Rapa MPs inhibited T1D, where 90% of mice survived for the duration of the study, while 90% of mice treated with empty MPs quickly reached humane endpoints (Fig. 8b, c ). However, Rapa MPs were also highly effective in preventing disease (Fig. 8b ). Together these data show in the NOD8.3 model of T1D, delivery of antigen/Rapa MPs or MPs only encapsulating Rapa is sufficient to inhibit disease when given at a timepoint close to disease induction. We hypothesized protection induced by Rapa MPs is transient, while inclusion of antigen with Rapa in MPs is necessary to promote durable tolerance. Fig. 8: Both Rapa MP and antigen/Rapa MPs inhibit T1D induction in therapeutic regimens, while co-encapsulation of antigen with Rapa is required for durable tolerance. a Schematic representation of therapeutic iLN treatment in the NOD8.3 model of T1D. e Survival curve for experiment detailed in a . c Individual blood glucose traces for mice in each group. d Schematic representation of iLN treatment with delayed disease induction in the NOD8.3 model of T1D. e Survival curve for experiment detailed in d . The number of surviving mice in each treatment group is shown in parenthesis in the legend. N = 10 mice for all groups in the therapeutic treatment regimen. N = 8 for all treatment groups in the delayed disease induction treatment regimen. Two-tailed log-rank (Mantel-Cox) was used for all pairwise comparisons between each treatment for survival curves in b and e . * p < 0.05, ** p < 0.01, *** p < 0.001, **** p < 0.0001. Source data are provided as a Source Data file. Intra-lymph node ( iLN ). Full size image To test whether the tolerance induced by MP treatment would be maintained even if T1D induction was performed at a much later timepoint after a single MP treatment, NOD mice were immunized 10 days before infusion of activated NOD8.3 T cells, and disease incidence was monitored daily (Fig. 8d ). Excitingly p31/Rapa MPs and NRP-V7/Rapa MPs significantly improved survival relative to vehicle and p31 MP treated mice (Fig. 8e ). The frequency of disease-free mice was more than doubled in both formulations combining antigen and Rapa compared to Rapa MP treatment. When benchmarking i.LN treatment of p31/Rapa MPs against soluble p31 and Rapa given i.p . at the 10 day timepoint (Supplementary Fig. 15a ), i.LN MPs provided superior efficacy (Supplementary Fig. 15b , c). Since antigen/Rapa MPs promoted durable tolerance compared to MPs encapsulating only Rapa, we next further investigated the phenotype of MP-induced antigen-specific T REG . MPs expand antigen-specific T REG with increased expression of markers of longevity Recent studies have demonstrated mTOR pathway inhibition during expansion of naïve T cells polarizes central memory phenotype among T REG , which display increased persistence in vivo [58] . Since antigen presentation after iLN treatment was prolonged (Fig. 6f–h ), we posited T REG responses polarized during mTOR inhibition may also be durable and create tolerogenic memory that has therapeutic significance in the context of autoimmune therapy. To test whether inclusion of Rapa in MPs enhances memory-like phenotype among self-reactive T REG , we first co-cultured DCs from NOD mice with BDC2.5 T cells in the presence of p31 MPs or p31/Rapa MPs. After 3 days T cells were stained for Foxp3 and markers characteristic of central memory T cells: CD44 + , CD62L + , and CCR7 (Supplementary Fig. 12 ). CD44 is a marker expressed by activated T cells; CD62L and CCR7 drive homing to LNs, where long-lived memory T cells persist [59] , [60] . Excitingly, co-cultures treated with p31/Rapa MPs increased the frequencies of T REG co-expressing CD62L and CD44 (Fig. 9a–c ), as well as CCR7 (Fig. 9d ). These in vitro results demonstrate inclusion of Rapa in MPs promotes antigen-specific T REG with central memory phenotypes. Fig. 9: MP treatment promotes expression of memory markers among antigen-specific T REG and durable tolerance in T1D. BDC2.5 T cell co-cultures were treated with p31 MPs or p31/Rapa MPs. a representative gating scheme to quantify co-expression of CD44 and CD62l among BDC2.5 T REG . Quantification of b CD44 + CD62L − and c CD44 + CD62L − frequencies T REG and ( d ) mean fluorescence intensity of CCR7 among BDC2.5 T REG . N = 3 for each sample. One-way ANOVA with Tukey’s post hoc test was used to compare all groups. Comparisons for p31 MP and p31/Rapa MPs at matched doses are indicated in plots. e Schematic representation of BDC2.5 T cell adoptive transfer experiment in panels f – k . N = 5 for each treatment group. f Representative flow cytometry plots showing BDC2.5 T cell frequency in treated LNs. Gating scheme for g p31 specific T REG and h co-expression of CD44 and CD62L, and expression of BCL-2 and CD127 among p31 specific T REG . Quantification of i co-expression of CD44 and CD62L, and expression of j BCL-2 and k CD127 among p31 specific T REG in treated LNs. Treated LNs were pooled for each mouse. One-way ANOVA with Tukey’s post hoc test was used to compare all groups. For all experiments mean ± s.d. is shown. * p < 0.05, ** p < 0.01, *** p < 0.001, **** p < 0.0001. Source data are provided as a Source Data file. Intra-lymph node ( iLN ). Full size image We next analyzed the effects of p31/Rapa MP treatment on the expression of central memory markers among antigen-specific T REG in vivo. NOD mice were immunized with p31/Rapa MPs, followed by adoptive transfer of BDC2.5 T cells (Fig. 9e ). 7 days after transfer, LNs were analyzed for expression of CD44, CD62L, as well as CD127 and Bcl-2 among antigen-specific Foxp3 + T REG (Fig. 9e , Supplementary Fig. 13 ) in treated LNs. CD127 is the receptor for IL-7, an important survival signal for memory T cells within LNs, and Bcl-2 preserves survival by inhibiting apoptosis [61] , [62] . LNs treated with p31/Rapa MPs retained significantly higher frequencies of antigen-specific T cells 1 week after adoptive transfer (Fig. 9f , Supplementary Fig. 14a , b ), and among these cells a higher number (Supplementary Fig. 14c ) and frequency of T REG (Fig. 9g , Supplementary Fig. 14d ). Excitingly, the number of antigen-specific T REG expressing CD44 + CD62L + (Fig. 9i ), Bcl-2 (Fig. 9j ) and CD127 (Fig. 9k ) was significantly higher in p31/Rapa MP treated LNs compared to all other treatment groups. In addition to absolute numbers, the frequency of Bcl-2 and CD127 expressing antigen-specific T REG was higher when comparing p31/Rapa MP treated LNs with p31 MP treated LNs (both treatment groups which expanded antigen-specific T cells) (Supplementary Fig. 14e–g ). Similar results were observed among the total antigen-specific CD4 T cell population (Supplementary Fig. 14h–j ). Thus, p31/Rapa MP treatment expands antigen-specific T REG in LNs and increases expression of markers associated with durability and regulatory memory. Taken together, Fig. 9 indicates LN treatment of MPs co-encapsulating islet antigen and Rapa expands antigen-specific T REG with a memory-like phenotype and supports co-delivery of antigen with Rapa is required for durable tolerance in T1D. Several possibilities may explain increased expansion of p31-specific T cells after treatment with p31/Rapa MP compared to p31 MP (Figs. 5 g and 9f ). Antigen-specific T cell proliferation may be more sustained after p31/Rapa MP treatment. In addition, reduced mTOR signaling during antigenic stimulation of T cells may drive a more durable phenotype for persistence and avoiding cell death. Previous reports have established mTOR inhibition to promote central memory phenotypes among cytotoxic T cells [63] , [64] , [65] ; however, only recently have the effects of mTOR inhibition on T REG memory phenotype [66] been explored. Recent work has demonstrated T REG in lymphoid tissue with low mTOR activity display increased markers of memory phenotype (Bcl2 high , CD62L high , KLRG1 low , PD-1 low ), lower levels of aerobic glycolysis, higher levels of oxidative phosphorylation and prolonged survival—all characteristics of long lived memory T cells [58] . While multiple reports have investigated co-delivering mTOR inhibitors with antigen to promote antigen-specific T REG [17] , [30] , [67] , this is the first report investigating the memory phenotype generated using this strategy. Here, p31/Rapa MP induced antigen-specific T REG expressed higher levels of markers associated with longevity (Fig. 9h, j, k ), and p31/Rapa MP treatment provided superior protection from T1D when disease was induced at a late timepoint following treatment (Fig. 8e ). Together these data support iLN treatment of tolerogenic MPs promote a durable and functional antigen-specific T REG response. Future studies will investigate the effects of p31/Rapa MPs on antigen-specific T REG survival and suppressive function over longer time periods. Here we demonstrate direct LN injection of MPs co-encapsulating Rapa with antigens targeted in autoimmune disease and alloimmune response is a potent therapeutic strategy to promote antigen-specific tolerance. MP treatment dramatically increased survival in models of T1D and islet transplantation mediated by both CD4 and/or CD8 pathology. Co-encapsulation of both MP components is necessary for optimal therapeutic efficacy. Mechanistically, inclusion of antigen is required to prime antigen-specific T cells in LNs, while Rapa functions to inhibit mTOR signaling during T cell priming. Excitingly, MPs expand T1D-relevant antigen-specific T REG in treated as well as distant LNs, creating tolerogenic microdomains in LNs that promote these regulatory immune responses. Thus, while drug delivery is localized, the suppressive and tolerogenic effects become systemic. From clinical safety and efficacy standpoints, the LN and its immunomodulatory depot could be removed in the case of localized toxicity, and the recipient avoids the systemic polypharmacy of current immunosuppression which almost universally relies on potent induction immunosuppression along with a cocktail of other agents, such as glucocorticoids, calcineurin inhibitors, and nuclei acid pathways inhibitors. Finally, MP treatment induced expression of markers associated with prolonged persistence and memory function among antigen-specific T REG and promoted durable tolerance in T1D. Together these data suggest a modular platform to promote lasting and selective tolerance in the context of T1D, potentially with reduced or eliminated side effects since not systemic or peripheral delivery is needed. Ethics All animal care and research was carried out using protocols approved and overseen by the University of Maryland and the University of Maryland IACUC committee (protocol R-Jan-22-04) in compliance with local, state, and federal guidelines. Animals All animal care and research was carried out using protocols approved and overseen by the University of Maryland IACUC committee in compliance with local, state, and federal guidelines. NOD (NOD/shiltJ), BDC2.5 (NOD.Cg-Tg(TcraBDC2.5,TcrbBDC2.5)1Doi/DoiJ), NOD8.3 (NOD.Cg-Tg(TcraTcrbNY8.3)1Pesa/DvsJ), TEa (B6.Cg-Tg(Tcra,Tcrb)3Ayr/J) C57BL/6J and BALB/c mice were purchased from The Jackson Laboratory. BDC2.5-thy1.1 mice were obtained from the Genetically Modified NOD Mouse Core Facility, Harvard Medical School, Pathology, NRB 1052 G, 77 Avenue Louis Pasteur, Boston, MA 02115. All NOD, C57BL/6, and BALBC mice used in studies were 8–10 weeks old. All NOD-thy1.1, NOD8.3 and TEa mice used in these studies were <3 months old. All NOD mice were non-diabetic at the start of each study. Only female mice were used in all studies. MP synthesis and characterization Degradable PLGA (Sigma Aldrich) MPs were synthesized as previously described [29] , [30] , [65] , [68] via double-emulsion. Briefly, an initial emulsion was generated by sonicating 80 mg 50:50 DL PLGA with 4 mg Rapa (LC labs) dissolved in 5 mL dichloromethane (Sigma-Aldrich) with 500 μL of water containing 1 mg of antigen. This initial emulsion was then homogenized with 40 mL water containing 1% w/v polyvinyl alcohol (Sigma) at 16,000 RPM for 3 min, and was allowed to evaporate overnight with stirring to allow evaporation of dichloromethane. MPs were then filtered through a 40 μm strainer (Corning Falcon) and collected via centrifugation at 5000 × g for 5 min at 4 °C. Supernatants were removed, and MPs were washed three times with 1 mL water. MPs were then resuspended in 1 mL water for in vitro and in vivo studies. Particle size was determined using an LA-950 laser diffraction analyzer (Horiba). To determine Rapa loading, a known mass of MPs was dissolved in dimethyl-sulfoxide (Sigma-Aldrich), and the absorbance at 278 nm was determined using UV/VIS spectrophotometry. Absorbance values were fit to a standard curve of known Rapa concentrations to calculate Rapa loading per mass of MPs. To determine peptide loading, Micro BCA Protein Assay Kit (Thermofisher Pierce) was used as previously described [30] , [69] . For preparation of fluorescently labeled MPs, 5 μL of DiR (Invitrogen) was dissolved with PLGA prior to the primary emulsion during MP synthesis. In vitro release kinetics To determine the release of microparticle cargo over time, a known mass of antigen-rapamycin microparticles was loaded into 10,000 kD MWCO dialysis tubing and placed in a 37 C 1× PBS sink condition in triplicate. At designated timepoints, an aliquot of MPs was removed from the dialysis tubing, lyophilized, then dissolved to a fixed MP concentration in 90% Acetonitrile in water. Remaining cargo in MPs was determined using high-performance liquid chromatography on a C18 column (XBridge TM BEH 300, C18, 3.5 μm, 2.1 × 50 mm). p31 antigen was detected at 220 nm. Proportion released was determined with respect to loading at time 0. For rapamycin release, p31-Rapa MPs were aliquoted in sink condition of PBS and incubated at 37 C. At each timepoint, aliquots were spun at 5000 × g for 5 min, aspirated and dissolved in 90% Acetonitrile in water. Concentration was determined via UV-Vis at 280 nm. Flow cytometry The following antibodies were used for flow cytometry: CD4 (clone GK1.5, diluted 1:300), Thy1.1 (clone OX7, diluted 1:200), CD8 (clone 53-6.7, diluted 1:300), CD62L (clone MEL-14, diluted 1:200), CD44 (clone IM-7, diluted 1:200), CD127 (clone SB/199, diluted 1:200), Bcl-2 (clone 3F11, diluted 1:100), Foxp3 (clone MF23, diluted 1:50), CD69 (clone H1.2F3, diluted 1:300), anti-s6 pS235/S236 (clone N7-548, diluted 1:10), IFNγ (clone XMG1.2, diluted 1:50), IL-17 (clone TC11-18H10, diluted 1:50). 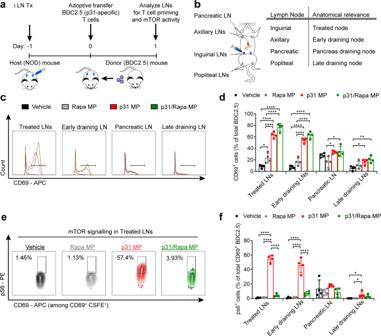Fig. 4: p31/Rapa MPs promote antigen-specific T cell priming while inhibiting mTOR in vivo. aSchematic representation of MP treatment and experimental readout for BDC2.5 T cell adoptive transfer experiment.bIllustration of lymph nodes collected and their anatomical relevance to treatment.cRepresentative flow cytometry traces anddquantification of CD69 expression among p31 specific T cells.eRepresentative flow cytometry traces of phosphorylated s6 among CD69+p31 specific T cells in treated LNs andfquantification in all LNs.N= 4 mice for all experiments, and paired LNs (i.e. inguinals, axillary, popliteal) were pooled for each mouse. The mean ±; s.d. is shown. One way ANOVA with Tukey’s post hoc test was used to compare each treatment within individual lymph nodes. *p< 0.05, **p< 0.01, ***p< 0.001, ****p< 0.0001. Source data are provided as a Source Data file. Intra-lymph node (iLN), phosphorylated ribosomal s6 protein (ps6). All antibodies for flow cytometry were purchased from BD biosciences. Mice were euthanized and lymph nodes collected and processed into single-cell suspension by mechanical dissociation through a 40μm cell strainer. Cells were washed once with PBS containing 1% w/v BSA (FACS buffer) and blocked with anti CD32/CD16 (BD, Clone 2.4G2, diluted 1:25) for 10 min at room temperature. Cells were then stained with surface marker antibodies for 20 minutes at room temperature. Cells were then washed two times with FACS buffer and were either analyzed immediately or stained for intracellular markers. For intracellular stains cells were fixed and permeabilized by incubating with fix/perm buffer from the Foxp3/Transcription factor staining buffer set (eBioscience) for 40 min at 4 degrees C. Cells were stained with antibodies against intracellular markers for 30 min at 4 degrees C, followed by two washes with perm/wash buffer. Cells were analyzed with a Canto II (BD) or FACSCelesta (BD). DAPI or LIVE/DEAD Fixable Viability Dye (Thermofisher) were used for cell viability. Flow cytometry data analysis was performed using FlowJo software (version 9, Treestar). In Vitro T cell co-cultures CD11c dendritic cells were isolated from mouse splenocytes using positive magnetic selection (Miltenyi) and were plated at 100,000 cells/well in 96 well plates. For co-cultures utilizing BDC2.5 or NOD8.3 T cells, dendritic cells (DCs) were isolated from NOD mice. For co-cultures utilizing Ea T cells, DCs were isolated from C57-BL6J mice. Following isolation, DCs were stimulated with 1 μg/mL lipopolysaccharide (LPS) to aid in T cell activation and treated with indicated doses of MPs for 24 h. T cells were then isolated from splenocytes using negative magnetic selection (Stemcell), labeled with 5 μL CSFE or CellTrace Violet (Thermofisher), and 300,000 T cells were co-cultured with MP-treated DCs for 3 days. CD4 + enrichment was used for BDC2.5 and Ea T cells, and CD8 + selection was used for NOD8.3 T cells. After 3 days, co-cultures were stimulated with cell stimulation cocktail (Thermofisher) in the presence of BFA (Biolegend) for 4 h, followed by surface and intracellular marker antibody staining and analysis flow cytometry to assess proliferation and determine T cell phenotype. Peptides p31 (YVRPLWVRME), Ea (ASFEAQGALANIAVDKA) and NRP-V7(KYNKANVFL) were synthesized by Genscript with purity >98%. Intra-lymph node injection iLN injection of mice was performed as previously described [29] , [30] , [65] , [68] , [69] . Briefly hair surrounding the injection site was removed using a mild depilatory cream, and mice were injected subcutaneously at the tail base with a tracer dye (Evan’s Blue). One day after tracer dye injection, both inguinal LNs were identified and injected with 1 mg of MPs, unless otherwise stated. MPs were suspended in 10 μL sterile water and injected iLN using a 31 g insulin syringe. Intra-peritoneal injection with soluble p31 and soluble rapamycin NOD mice were injected i.p at the indicated treatment times and doses with soluble p31 and soluble rapamycin in 100 μL of 5% DMSO in PBS. Diabetes induction through NOD8.3 T cell adoptive transfer 8 week old female NOD mice were immunized iLN with indicated MP treatments. Splenocytes from NOD8.3 mice were stimulated with 1 μM NRP-V7 peptide at 2 × 10 6 cells/mL for 3 days, washed with PBS, and injected i.v . into host NOD mice at 15 × 10 6 cells/mouse. Blood glucose was monitored daily following T cell infusion, and mice were considered diabetic at a blood glucose level >250 mg/dL. Islet transplantation studies 8–10 week old C57BL/6 mice were induced with diabetes by intra-peritoneal injection of 180 mg/kg Streptozotocin. Islets were implanted and lymph nodes were injected with indicated treatments on the day host mice became diabetic. The time interval (Δt) between Streptozotocin and islet transplantation was 7–14 days for all mice in the study. To collect allogenic islets, BALB/c mice were euthanized and the common bile duct was injected with 3 mL cold Hanks’ buffer containing 1.5 mg/mL of collagenase-P (Roche Diagnostics, Indianapolis, IN). Pancreata was surgically excised and digested at 37 °C for 15 min. The digested pancreas was disrupted by vigorous shaking, and the suspension was washed twice with RPMI 1640 containing 10% fetal bovine serum. Pancreatic islet separation was performed by centrifugation on a discontinuous Ficoll (Sigma) gradient of 11%, 21%, 23%, and 25%. Islets were picked from the second layer, and 400 islets were transplanted beneath the renal capsule of host mice. Blood glucose was monitored daily, and mice were euthanized after two consecutive readings of blood glucose >300 mg/dL. BDC2.5 T cell adoptive transfer studies 8–10 week old female NOD mice were immunized iLN with indicated MP treatments. One day following iLN treatment, BDC2.5 T cells were isolated from splenocytes of BDC2.5 mice BDC2.5-thy1.1 mice using CD4 negative magnetic selection (Stemcell) per the manufacturer’s instructions and were adoptively transferred to host NOD mice T cells/mouse. In studies using BDC2.5 T cells, cells were labeled with CSFE prior to adoptive transfer. At indicated times following T cell transfer, host mice were sacrificed and LNs were processed and analyzed by flow cytometry. BDC2.5 T cells were identified based on CSFE signal when using BDC2.5 T cells or the expression of thy1.1 when using BDC2.5-thy1.1 T cells. In vivo imaging Imaging of indicated surgically excised LNs was performed using a Perkin-Elmer IVIS Spectrum in vivo imaging system. DiR (Thermo) Fluorescent MPs were synthesized using MP double emulsion described with 0.4 mg DiR added to the organic polymer solution. Animals were injected iLN with MPs as described with either empty (non-fluorescent), or Vehicle MPs. 2 and 4 days following iLN injection, mice were euthanized and LNs were excised and imaged. Exposure times and lamp settings were determined from single-fluorophore controls. Image analysis was performed using Living Image Software (Perkin Elmer) and quantitative analysis was done using doing region of interest (ROI) analysis of total radiant efficiency. Number of mice and LNs imaged are indicated in figure legends. Immunohistochemistry and histology The following primary antibodies were used for immunohistochemistry diluted 1:200: ERTR7 (scbt, clone sc-73355), CD11c (BD, clone HL3), Laminin alpha 4 (Novus Bio, clone 775830), laminin alpha 5 (Novus Bio, polyclonal), Foxp3 (ThermoFisher, clone NRRF-30), Y-Ae (scbt, clone sc-32247). For immunohistochemistry, LNs and spleens were frozen with OCT compound (Scigen Tissue-Plus). Frozen sections were cut at 6μm, fixed with cold acetone, blocked with 5% goat or donkey serum (Jackson ImmunoResearch, West Grove, PA) and incubated with the indicated antibodies and DAPI. Samples were incubated with secondary antibodies diluted 1:400 for 1 h (Rabbit IgG, Goat polyclonal, Jackson Immunoresearch; Rat IgG Goat Polyclonal, Jackson Immunoresearch; Rabbit IgG, Donkey Polyclonal, Jackson Immunoresearch; Rat IgM, Goal Polyclonal Jackson Immunoresearch). Samples were further processed as described previously [45] , [46] , [56] . Images were acquired with a Nikon Eclipse 700 (Nikon, Melville, NY, USA) and analyzed with Volocity image analysis software (version 4.7.2) Perkin Elmer, Waltham, MA). The positive staining area percentage was quantified based on at least three independent experiments with 3 sections per LN and 3–5 fields/section. Number of mice are indicated in figure legends. Statistics and reproducibility Analyses were carried out with Graphpad Prism (version 9.3.1). The specifics of statistical tests for each experiment and the number of replicates are detailed in figure legends. 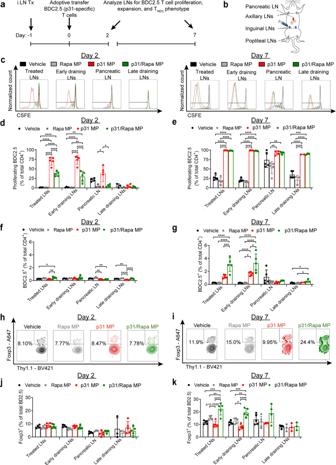Fig. 5: p31/Rapa MPs expand antigen-specific TREGin treated and untreated LNs. aSchematic representation of MP treatment and experimental readout for BDC2.5 T cell adoptive transfer experiment.bIllustration of LNs collected and analyzed.cRepresentative flow cytometry traces and quantification of p31 specific T cell proliferation atdday 2 andeday 7. Quantification of p31 specific T cell frequency atfday 2 andgday 7. Representative flow cytometry traces showing Foxp3 expression among p31 specific T cells in treated LNs athday 2 andiday 7. Quantification of Foxp3 expression among p31 specific T cells atjday 2 andkday 7 in each LN analyzed.N= 5 mice for all groups in all experiments, and paired LNs were pooled for each mouse. The mean ±  s.d. is shown. For all comparisons in this figure between mice treated with different treatments, One-way ANOVA with Tukey’s post hoc test was done between all treatment groups within each individual LN. All comparisons between the Rapa MP and p31/Rapa MP treatment groups among different tissues were also done using One way ANOVA with Tukey’s post hoc test, and thepvalues from this analysis are listed in Supplemental Table2. *p< 0.05, **p< 0.01, ***p< 0.001, ****p< 0.0001. Source data are provided as a Source Data file. Intra-lymph node (iLN). Error bars in all panels represent the mean ± standard deviation and p values ≤ 0.05 were considered significant with levels of significance were defined as * p < 0.05, ** p < 0.01, *** p < 0.001, **** p < 0.0001. For comparisons of more than two groups, one-way ANOVA with Tukey’s post test was performed. For comparisons of two groups, two-tailed Welch’s t test was performed. For T1D and allogenic islet transplantation survival studies, two-tailed log-rank (Mantel-Cox) was used for all pairwise comparisons between each treatment for survival curves. For experiments using immunohistochemistry and histology, representative images of data from two similar experiments are shown. 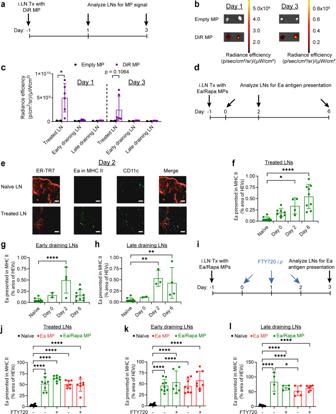Fig. 6: Ea is presented in treated and untreated LNs after Ea/Rapa MP treatment. aSchematic representation of experiment in panelsb–d.bIVIS images of excised treated LNs.cQuantitation of DiR MP signal in excised LNs. Two-tailed Welch’sttest was used to compare both treatment groups within individual lymph nodes at each time point. Individual LNs were used as single data points. Mean ± s.d. is shown.N= 3 mice for DiR MP treatment groups andN= 1 mouse for empty MP treatment group at each timepoint. Each LN is represented as an individual data point.dSchematic representation of experiment in panelsf–i.eRepresentative immunofluorescent images of LNs stained with ER-TR7, CD11c, YAe; Scale bar = 50 μm. Quantification of Ea presentation in MHC-II (YAe) inftreated,gearly-draining andhlate-draining LNs.N= 2 mice for each timepoint, with 2 or 3 sections per LN. One way ANOVA with Dunnett’s post hoc test was used to compare percent YAe area to the naive control at each timepoint.iSchematic representation of experiment in panelsk–m. Quantification of Ea presentation in MHC-II injtreated,kearly-draining andllate-draining LNs after FTY720 treatment. One-way ANOVA with Tukey’s post hoc test was used to compare each group.N= 2 mice for each timepoint, with 2 or 3 sections per LN. Mean ± s.d. is shown for each sample in each experiment. *p< 0.05, **p< 0.01, ***p< 0.001, ****p< 0.0001. Source data are provided as a Source Data file. Intra-lymph node (iLN). 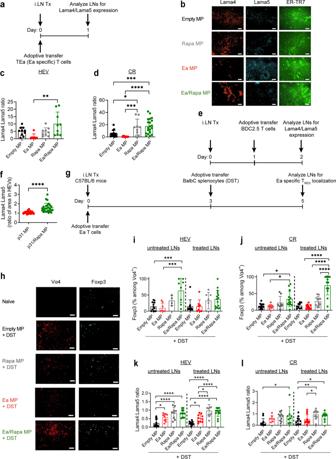Fig. 7: MP treatment promotes development of tolerogenic microdomains in LNs. aSchematic representation of experiment in panelsb–d.bRepresentative immunofluorescence images of treated LNs stained for laminin α4, laminin α5, ER-TR7, and DAPI are shown; Scale bar = 50 μm. Quantification of ratio of laminin α4 to laminin α5 inchigh endothelial venules anddcortical ridges in treated LNs.N= 4 mice for each treatment group with 2 or 3 sections per LN. One-way ANOVA with Tukey’s post hoc test was used to compare treatment groups.eSchematic representation of experiment in panelf.fRatio of laminin α4 to laminin α5 in high endothelial venules of LNs.N= 4 mice for each treatment group with 2 or 3 sections per LN. Two-tailed Welch’sttest was used to compare groups, and inguinal, axillary and pancreatic LNs were pooled for each treatment group.gSchematic representation of experiments in panelsi–l.hRepresentative immunofluorescence images showing Foxp3 expression among antigen-specific T cells in treated LNs. The naïve group did not receive adoptive transfer of Ea T cells. DAPI (Blue) and ER-TR7 (Cyan) are included in the merge: Scale bar = 50 μm. LNs were stained for Foxp3, Vα4 T cell receptor clonotype, ER-TR7, and DAPI. Representative merged images are show in Supplementary Fig.10. Quantification of Foxp3 expression among antigen-specific T cells inihigh endothelial venules (HEV) andjcortical ridges (CR). Quantification of ratio of laminin α4 to laminin α5 inkhigh endothelial venules andlcortical ridges in treated and untreated LNs.N= 4 mice for each treatment group with 2 or 3 sections per LN. Iliac LNs were used as untreated LNs. One-way ANOVA with Tukey’s post hoc test were used to compare each treatment group within individual lymph nodes in each region of the LN analyzed. For all experiments mean ± s.d. is shown. *p< 0.05, **p< 0.01, ***p< 0.001, ****p< 0.0001. Source data are provided as a Source Data file. Intra-lymph node (iLN). 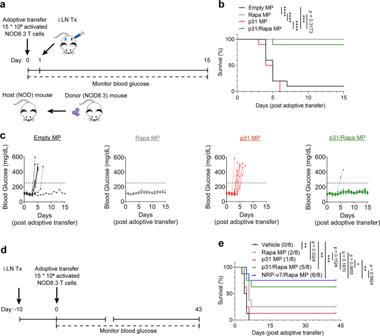Fig. 8: Both Rapa MP and antigen/Rapa MPs inhibit T1D induction in therapeutic regimens, while co-encapsulation of antigen with Rapa is required for durable tolerance. aSchematic representation of therapeuticiLNtreatment in the NOD8.3 model of T1D.eSurvival curve for experiment detailed ina.cIndividual blood glucose traces for mice in each group.dSchematic representation of iLN treatment with delayed disease induction in the NOD8.3 model of T1D.eSurvival curve for experiment detailed ind. The number of surviving mice in each treatment group is shown in parenthesis in the legend.N= 10 mice for all groups in the therapeutic treatment regimen.N= 8 for all treatment groups in the delayed disease induction treatment regimen. Two-tailed log-rank (Mantel-Cox) was used for all pairwise comparisons between each treatment for survival curves inbande. *p< 0.05, **p< 0.01, ***p< 0.001, ****p< 0.0001. Source data are provided as a Source Data file. Intra-lymph node (iLN). 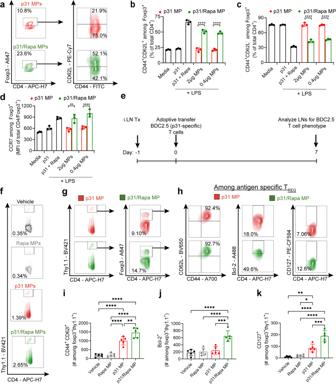Fig. 9: MP treatment promotes expression of memory markers among antigen-specific TREGand durable tolerance in T1D. BDC2.5 T cell co-cultures were treated with p31 MPs or p31/Rapa MPs.arepresentative gating scheme to quantify co-expression of CD44 and CD62l among BDC2.5 TREG. Quantification ofbCD44+CD62L−andcCD44+CD62L−frequencies TREGand (d) mean fluorescence intensity of CCR7 among BDC2.5 TREG.N= 3 for each sample. One-way ANOVA with Tukey’s post hoc test was used to compare all groups. Comparisons for p31 MP and p31/Rapa MPs at matched doses are indicated in plots.eSchematic representation of BDC2.5 T cell adoptive transfer experiment in panelsf–k.N= 5 for each treatment group.fRepresentative flow cytometry plots showing BDC2.5 T cell frequency in treated LNs. Gating scheme forgp31 specific TREGandhco-expression of CD44 and CD62L, and expression of BCL-2 and CD127 among p31 specific TREG. Quantification ofico-expression of CD44 and CD62L, and expression ofjBCL-2 andkCD127 among p31 specific TREGin treated LNs. Treated LNs were pooled for each mouse. One-way ANOVA with Tukey’s post hoc test was used to compare all groups. For all experiments mean ± s.d. is shown. *p< 0.05, **p< 0.01, ***p< 0.001, ****p< 0.0001. Source data are provided as a Source Data file. Intra-lymph node (iLN). Reporting summary Further information on research design is available in the Nature Portfolio Reporting Summary linked to this article.